Regulatory change atPhysalis Organ Size 1correlates to natural variation in tomatillo reproductive organ size The genetic basis of size variation in the reproductive organs of tomatillo ( Physalis philadelphica ) is unknown. Here we report that the expression levels of the gene Physalis Organ Size 1 ( POS1 ) are positively associated with size variation in P. philadelphica reproductive organs such flowers, berries and seeds. POS1 knockdown results in smaller flowers and berries with smaller cells as compared with their wild-type counterparts. Conversely, POS1 overexpression promotes organ size without increasing the cell number. The first introns of the POS1 alleles from the large, intermediate and small tomatillo groups contain one, two and three 37-bp repeats, respectively. Furthermore, our results show that copy variation of repeats in the first intron of POS1 alleles results in differential expression of this gene. Thus, co-variation in tomatillo reproductive organ sizes can be attributed to the novel regulatory variation in POS1 . Plant reproductive organs include floral organs, seeds and fruits. The developmental genetic regulators specifying their organ identity are well characterized [1] , [2] , [3] . However, it is important to elucidate the genetic basis regulating organ size, especially the fruits and seeds [4] , [5] , [6] . The fruit is the main commodity of important Solanaceous crops, such as tomato ( Solanum lycopersicum ), eggplant ( Solanum melongena ) and pepper ( Capsicum sp. ). The control of berry size is a prime breeding target to enhance yield in these crops. Nearly 30 quantitative trait loci (QTLs) accounting for fruit size were detected in tomato [7] , [8] , [9] , [10] , eggplants and pepper [9] , [11] , [12] . However, most of them have not been cloned, and little is known about the nature of the encoded gene products. So far, only three of these QTLs have been identified in tomato. Fruit weight 2.2 ( FW2.2 ) was the first QTL characterized in plants via a map-based cloning approach [13] . A mutation in the FW2.2 promoter resulted in fruit enlargement via heterochronic expression of the gene during fruit development [13] , [14] , [15] . FW2.2 is a plasma membrane-anchored protein, which is involved in the cell cycle pathway for ovary size control [16] . Another two cloned loci namely fasciated ( fas ) and locule number ( lc ) mainly control the locule number of ovary [17] , [18] . FAS encodes a YABBY-like transcription factor, and the mutation that increases the locule number and fruit weight resulted from an insertion knocking out the gene [17] . The molecular nature of LC is two single-nucleotide polymorphisms located ~1,200 bp downstream of the stop codon of the tomato orthologue of WUSCHEL , a gene encoding a homeodomain protein regulating stem cell fate in plants [18] . Convergent domestication resulting from mutations and selection at the common loci was observed in members of the family Solanaceae including tomato, eggplants and pepper [9] , [11] , [12] . Physalis has emerged as a new leading Solanaceous horticultural crop and as a new plant model for ecology, evolution and development [19] , [20] . The genus Physalis features a fruiting calyx shaped like a Chinese lantern, also called the inflated calyx syndrome (ICS), a novelty of the floral calyx formed after fertilization that is controlled by several MADS-box transcription factors [19] , [21] , [22] . Unlike Solanum and Capsicum species, Physalis has distinguished fruit morphology owing to the accessory ICS trait. The fruiting calyces and the berries of a few Physalis species have curative and culinary usages [23] ; however, the berry inside is still an important agronomic trait. Physalis philadelphica (tomatillo) is one of the few Physalis species used as a crop for berries. Tomatillos originated in Mexico and have been cultivated since pre-Columbian times (800 BC) by the Aztecs from its wild types (WTs) that grew along the Pacific coast, from California to Guatemala [23] , [24] , [25] . The berry size varies markedly among various tomatillo cultivars/accessions ( Fig. 1 ); however, the genetic basis underlying the variation is yet not known. Transcriptome-wide screens showed that the expression of Pp30 , putatively encoding an APETALA2 (AP2)-like transcription factor is associated with flower and berry size in tomatillo. Furthermore, this gene was proposed to be a valuable candidate gene for the evolution of natural variation of the reproductive organ size in Physalis [20] . 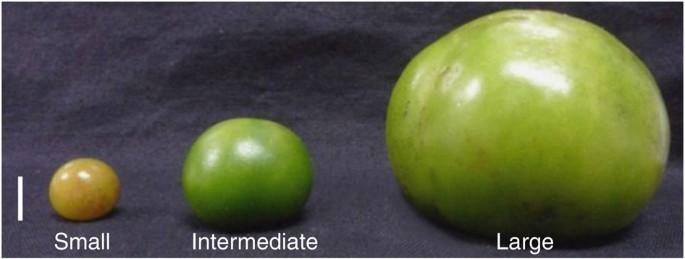Figure 1: Variation of berry size in tomatillos. A berry phenotype of tomatillos (from left to right) is from three distinct groups with small, intermediate and large berry size. The lantern-like fruiting calyces were removed to show the berries. Scale bar, 1 cm. The details of reproductive organ-size variation inPhysalis philadelphicaare available inSupplementary Fig. 1;Supplementary Table 1. Figure 1: Variation of berry size in tomatillos. A berry phenotype of tomatillos (from left to right) is from three distinct groups with small, intermediate and large berry size. The lantern-like fruiting calyces were removed to show the berries. Scale bar, 1 cm. The details of reproductive organ-size variation in Physalis philadelphica are available in Supplementary Fig. 1 ; Supplementary Table 1 . Full size image In the present study, we characterize this locus, hereafter referred to as Physalis Organ Size 1 ( POS1 ), and use multiple approaches to confirm its role as a positive regulator of cell expansion. We further survey the naturally occurring allelic variations to establish the molecular basis for the observed organ-size variation. Our data reiterate that altered gene expression, due to a regulatory change in introns during evolution, can affect the plant morphology. POS1 expression is associated with organ sizes in tomatillos After 3-year field tests, 37 accessions of P. philadelphica were grouped as those having large, immediate and small reproductive organs ( Supplementary Fig. 1 ; Supplementary Table 1 ). 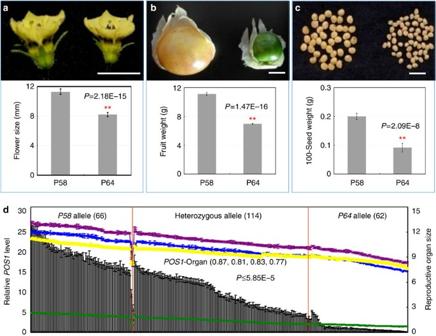Figure 2:Genetic linkage and association analyses of the tomatilloPOS1locus, gene expression and reproductive organ sizes in the F2population. (a–c) Size variations of reproductive organs between P58 and P64 ofP. philadelphica. (a) Flowers (b) fruits and (c) seeds. Scale bar, 1 cm. Error bars are the s.d. AllP-values are based on the two-tailedt-test. The ** indicate a significant difference (P<0.01) between P58 and P64. (d) Association and linkage ofPOS1locus, gene expression and reproductive organ size. Total RNA from mature flowers was subjected to qRT–PCR analyses. ThePFACTINgene was used as an internal control. Three independent biological replicates were used. Error bars are s.d. Black column,POS1expression; yellow line, flower size (mm); purple line, berry weight (g); blue line, berry volume (cm3); green line, 100-seed weight. Correlation coefficients forPOS1expression with these traits in order (flower size, berry weight, berry volume and 100-seed weight) are shown in parenthesis. We found significant positive correlations among the size variations of these organs ( Supplementary Table 2 ). To avoid the effects of polyploidy on the organ size, we first evaluated the chromosome number of these tomatillo accessions and found that they were all likely diploid and had chromosomes approaching 24 ( Supplementary Table 1 ). Thus, polyploidy does not play a role in the huge variation of reproductive organ sizes. We checked for POS1 messenger RNA (mRNA) accumulation in mature flowers and berries from each accession 10 days post fertilization to establish a link between POS1 and variation in organ size. A significant correlation was established between POS1 expression levels and organ size ( Supplementary Fig. 1 ; Supplementary Table 2 ). Higher expression of POS1 corresponded to a bigger organ size while a lower expression entailed a smaller organ size [20] . Thus, POS1 may positively regulate reproductive organ size of tomatillo in a dosage-dependent manner. Next, we confirmed the role of the POS1 alleles in a segregating population through gene expression–organ size association analysis. The final size of flowers ( Fig. 2a ), fruits ( Fig. 2b ) and seeds ( Fig. 2c ) of the tomatillo accession P64 was significantly smaller than that of the accession P58. Thus, the two tomatillo accessions were chosen as parents to construct a segregating population. Reciprocal crosses showed that the organ size was a maternally inherited trait such as fruits and seeds ( Supplementary Fig. 2a–e ). The F 2 population with 242 progeny from a cross of P58 (♀) and P64 (♂) was analysed. Two molecular genetic markers (the MADS-box gene 2 from P. floridana ( MPF2 ) [19] - and the POS1 originated) were used to evaluate segregation. Both markers showed polymorphisms between the two parents P58 and P64 ( Supplementary Fig. 2f ), and they segregated in the population with a ratio of P58: P58-P64: P64 as 1:2:1 ( χ 2 =0.02, P >0.05 for POS1 (66:114:62); χ 2 =0.01, P >0.05 for MPF2 (60:117:65)). Size variation of flowers, berries and seeds conformed to a normal distribution in the segregating population ( Supplementary Fig. 2g ). Correlation coefficients among these organ-size variations were >0.97 ( P ≤1.53E−6, Supplementary Fig. 2h ), suggesting a shared genetic basis for the size co-variation of these organs in P. philadelphica . Figure 2: Genetic linkage and association analyses of the tomatillo POS1 locus, gene expression and reproductive organ sizes in the F 2 population. ( a – c ) Size variations of reproductive organs between P58 and P64 of P. philadelphica . ( a ) Flowers ( b ) fruits and ( c ) seeds. Scale bar, 1 cm. Error bars are the s.d. All P -values are based on the two-tailed t -test. The ** indicate a significant difference ( P <0.01) between P58 and P64. ( d ) Association and linkage of POS1 locus, gene expression and reproductive organ size. Total RNA from mature flowers was subjected to qRT–PCR analyses. The PFACTIN gene was used as an internal control. Three independent biological replicates were used. Error bars are s.d. Black column, POS1 expression; yellow line, flower size (mm); purple line, berry weight (g); blue line, berry volume (cm 3 ); green line, 100-seed weight. Correlation coefficients for POS1 expression with these traits in order (flower size, berry weight, berry volume and 100-seed weight) are shown in parenthesis. Full size image Furthermore, the progeny with homozygous POS1 -P58 alleles had higher expression levels of this gene while homozygous POS1 -P64 alleles had lower expression levels. The progeny harbouring heterozygous alleles had gene expression levels that varied between homozygous POS1 -P64 and POS1 -P58 alleles ( Fig. 2d ). The distribution of the POS1 expression trait in the segregating population also complied with the characteristics of the quantitative traits ( Supplementary Fig. 2g ). The expression levels co-segregated with the POS1 allele ( χ 2 =6.66, P <0.01), but were independent of the MPF2 allele ( χ 2 =0.59, P >0.05), suggesting that a master regulatory cis -element near or within the POS1 locus was responsible for variation in the expression trait. There was a clear association between POS1 expression and the size of reproductive organs ( Fig. 2d ), and the expression variation of POS1 could account for 69.8, 63.1 and 61.3% of the size variation in berries, floral organs and seeds, respectively, between P58 and P64. Therefore, POS1 expression is probably involved in the control of reproductive organ size in tomatillos. Next, we monitored the expression of different POS1 alleles during flower and fruit development. mRNA expression experiments were conducted using quantitative reverse transcriptase PCR (qRT–PCR). POS1 was predominantly expressed in the reproductive organs, preferentially in ovaries and developing berries in P. philadelphica (P58, P64 and P59 accessions) and P. floridana P106 ( Fig. 3a ), and its expression was upregulated during berry development [20] ( Supplementary Fig. 3a ). POS1 genes from the four Physalis accessions showed similar expression profiles during flower and fruit development; however, different dosage in different accessions appeared to be positively correlated to reproductive organ size. A further mRNA in situ hybridization with an antisense probe in P. floridana (P106) showed that POS1 was restricted to floral tissues from floral initiation to organ formation. POS1 mRNA was localized in floral meristems, floral organ primordia and organs such as the calyx, corolla, stamen and ovary in the early-flower development, in placental tissues, ovules, the tissues surrounding the ovules at later stages and in developing seeds and berries ( Fig. 3b–i ). Furthermore, no expression signal was detected in either apical meristem or leaf buttress/primordia ( Fig. 3j ). A sense probe was hybridized as control ( Supplementary Fig. 3b–h ). These results further suggest the role of POS1 genes in flower and fruit development. 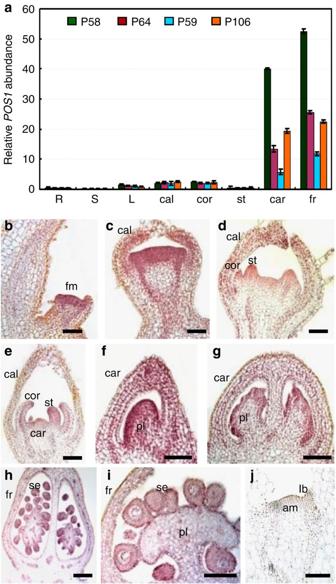Figure 3:Differential floral and fruit expressions of thePOS1genes inPhysalis. (a) qRT–PCR analyses of tissue-specific accumulation of thePOS1genes in P58, P64, P59 and P106. R, root; S, stem; L, leaf; cal, calyx; cor, corolla; st, stamen; car, carpel; fr, fruit. Green column, P58; purple column, P64; blue column, P59; red column, P106. Three independent biological samples were used. ThePFACTINgene was used as an internal control. The expression in P64 was set as 1. Error bars are s.d. (b–j) RNAin situhybridizations. Tissue sections were hybridized with aPOS1-P106 antisense RNA probe. (b) Early development with initiation of calyx primordia. (c) Early development before initiation of corolla primordia. (d,e) Early development before initiation of carpel primordia. (f–i) Late-stage development. (f–h) Longitudinal section of an ovary and a berry. (i) Cross-section of a berry. (j) NoPOS1expression was detected in the stem apex. Hybridizations with aPOS1-P106 sense RNA probe as a control at different developmental stages are presented inSupplementary Fig. 3b–h. fm, floral meristem; cal, calyx primordia; cor, corolla primordia; st, stamen primordia; car, carpel primordia; pl, placenta; fr, fruit; se, seed; am, apical meristem; lb, leaf buttress. Scale bar, 100 μm. Figure 3: Differential floral and fruit expressions of the POS1 genes in Physalis . ( a ) qRT–PCR analyses of tissue-specific accumulation of the POS1 genes in P58, P64, P59 and P106. R, root; S, stem; L, leaf; cal, calyx; cor, corolla; st, stamen; car, carpel; fr, fruit. Green column, P58; purple column, P64; blue column, P59; red column, P106. Three independent biological samples were used. The PFACTIN gene was used as an internal control. The expression in P64 was set as 1. Error bars are s.d. ( b – j ) RNA in situ hybridizations. Tissue sections were hybridized with a POS1 -P106 antisense RNA probe. ( b ) Early development with initiation of calyx primordia. ( c ) Early development before initiation of corolla primordia. ( d , e ) Early development before initiation of carpel primordia. ( f – i ) Late-stage development. ( f – h ) Longitudinal section of an ovary and a berry. ( i ) Cross-section of a berry. ( j ) No POS1 expression was detected in the stem apex. Hybridizations with a POS1 -P106 sense RNA probe as a control at different developmental stages are presented in Supplementary Fig. 3b–h . fm, floral meristem; cal, calyx primordia; cor, corolla primordia; st, stamen primordia; car, carpel primordia; pl, placenta; fr, fruit; se, seed; am, apical meristem; lb, leaf buttress. Scale bar, 100 μm. Full size image The role of variation in POS1 expression in Physalis reproductive organ-size variation was investigated in transgenic P. floridana (P106) lines. Altering POS1 expression changes P. floridana organ sizes A 480-bp POS1 -P106-specific complementary DNA (cDNA) fragment was introduced into the tobacco rattle virus (TRV)-based virus-induced gene silencing (VIGS) to downregulate POS1 -P106. As a result of this, the size of the population of 100 randomly harvested mature flowers could be classified according to size into three grades (V-I, V-II and V-III) in the VIGS population ( Supplementary Fig. 4a ). Mature floral organ-size variation in grade I (V-I) was comparable to that in the WT. However, the size of floral organs, that is, the calyx, corolla, stamen and ovary in grades II (V-II) and III (V-III) was significantly smaller ( P ≤0.04) than that of the WT ( Fig. 4a ; Supplementary Fig. 4b–d ). In comparison with WT, organ size in grades I, II and III was decreased by 8.14–40.86% ( Supplementary Table 3 ). Downregulation of POS1 expression also affected mature berry size. Although berry size in grade I statistically remained the same as that of WT (1.26±0.16 g), grade II and grade III berries showeda marked reduction in weight and volume (19.70–42.74% lower than WT) ( P <0.05, Fig. 4b ; Supplementary Fig. 5 ; Supplementary Table 3 ). We randomly selected eight flowers/berries from the WT as well as each grade in the POS1 -VIGS population and subjected the samples to qRT–PCR analyses. POS1 expression variation in grade I flowers/berries was equivalent to that in WT flowers/berries while it was significantly lower in grade II and III flowers/berries. This can be attributed to the gene silencing efficiencies by VIGS within a plant; however, the correlation coefficient of gene expression with flower/berry size was around 0.90 ( P ≤1.09E−4, Supplementary Figs 4e and 5d ). Furthermore, the ICS became smaller in grades II and III ( Supplementary Fig. 5a ). PFCRF7 and PFCRF8 of Physalis are the closest homologues of POS1 ( Supplementary Fig. 6a ). We isolated these two homologues to substantiate the specificity of downregulating POS1. The expressions of PFCRF7 and PFCRF8 were not statistically altered in the POS1 -VIGS organs ( Supplementary Figs 4a and 5a ). Moreover, the reproductive organ size was not significantly altered in the controls, wherein both PfPDS and PfP12 were silenced by the same VIGS approach and cultivating conditions ( Supplementary Fig. 6b–f ). 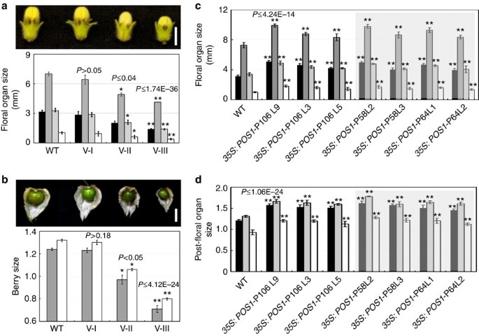Figure 4:AlteringPOS1expression regulates reproductive organ size inPhysalis. (a,b) SilencingPOS1decreased flower and berry size. (a) The above images show an overall reduction in flower size of three different degrees of phenotypic variation and gene expression levels. From left to right: WT, V-I, V-II and V-III. Scale bar, 5 mm. The below graph quantified the size variation in floral organs. From left to right: calyx (black column), corolla (dark-grey column), stamen (light-grey column) and carpel (empty column). (b) The above images show a reduction in berry size. From left to right: WT, V-I, V-II and V-III. Scale bar, 1 cm. The below graph quantified the berry size. Berry weight (g), grey column; berry volume (cm3), empty column. (c,d) OverexpressingPOS1cDNA alleles increased the reproductive organ size. (c) Quantification of floral organ size. Black column, calyx size (mm); dark-grey column, corolla size (mm); light-grey column, stamen size (mm); empty column, ovary size (mm). (d) Quantification of berry and seed size. Berry weight (g), black column; berry volume (cm3), grey column; 100-seed weight (g), empty column. Two tomatillo allelesPOS1-P58 andPOS1-P64 were also overexpressed inP. floridana, and similar phenotypic variations were observed (grey section incandd). Error bars are s.d. AllP-values are based on the two-tailedt-test. Compared with WT, the * indicates a significant difference (P<0.05), and the ** indicate a significant difference (P<0.01). For images, seeSupplementary Figs 8–10. Figure 4: Altering POS1 expression regulates reproductive organ size in Physalis . ( a , b ) Silencing POS1 decreased flower and berry size. ( a ) The above images show an overall reduction in flower size of three different degrees of phenotypic variation and gene expression levels. From left to right: WT, V-I, V-II and V-III. Scale bar, 5 mm. The below graph quantified the size variation in floral organs. From left to right: calyx (black column), corolla (dark-grey column), stamen (light-grey column) and carpel (empty column). ( b ) The above images show a reduction in berry size. From left to right: WT, V-I, V-II and V-III. Scale bar, 1 cm. The below graph quantified the berry size. Berry weight (g), grey column; berry volume (cm 3 ), empty column. ( c , d ) Overexpressing POS1 cDNA alleles increased the reproductive organ size. ( c ) Quantification of floral organ size. Black column, calyx size (mm); dark-grey column, corolla size (mm); light-grey column, stamen size (mm); empty column, ovary size (mm). ( d ) Quantification of berry and seed size. Berry weight (g), black column; berry volume (cm 3 ), grey column; 100-seed weight (g), empty column. Two tomatillo alleles POS1 -P58 and POS1 -P64 were also overexpressed in P. floridana , and similar phenotypic variations were observed (grey section in c and d ). Error bars are s.d. All P -values are based on the two-tailed t -test. Compared with WT, the * indicates a significant difference ( P <0.05), and the ** indicate a significant difference ( P <0.01). For images, see Supplementary Figs 8–10 . Full size image We also overexpressed the POS1 alleles ( POS1- P106, POS1 -P58 and POS1 -P64) in P. floridana via Agrobacterium -mediated transformation driven by a 35S promoter. Multiple, independent T 1 transgenic lines were regenerated, and lines with obvious phenotypic variations were further characterized in their T 2 progeny ( Supplementary Fig. 7 ). In comparison with WT, the size of all reproductive organs was increased ( Fig. 4c,d ; Supplementary Fig. 8a–e ). Mature floral organs, including the calyx, corolla, stamen and carpel became significantly larger in these transgenic plants ( P ≤4.24E−14) ( Fig. 4c ). The increase in the size of reproductive organs was 18.97–43.91% over the WT flowers ( Supplementary Table 3 ). The size of the mature berry and seed also increased significantly ( P ≤1.06E−24) by 21.37–29.75% compared with the WT organs ( Fig. 4d ; Supplementary Fig. 8f–i ; Supplementary Table 3 ). The overexpressed lines showed a larger ICS as compared with the WT plants ( Supplementary Fig. 8f ). POS1 -P58- and POS1 -P64-overexpressing transgenic lines of P. floridana showed similar phenotypic variations ( Fig. 4c,d ; Supplementary Figs 9 and 10 ). However, the seed number per berry was not affected in all of the POS1 overexpressors ( P ≥0.06, Supplementary Fig. 11 ). Therefore, a higher expression of POS1 alleles induced a bigger organ size while silencing this gene resulted in reduced organ size. POS1 gene activity promotes cell expansion We further examined the POS1 effects on cell division and cell expansion. For this, we investigated the epidermal cells of the mature floral organs including calyx, corolla, stamen, ovary and the median transverse sections of berries 3 days after fertilization ( Fig. 5 ; Supplementary Fig. 3 ). In the POS1 -P106-silenced flowers, the epidermal cells of floral organs ( Fig. 5a ; Supplementary Fig. 12a–e ) and the cells in the exocarp, mesocarp and placenta ( Fig. 5b ; Supplementary Fig. 12f–h ) were significantly smaller in grades II and III plants as compared with WT and grade I ( P ≤0.04). Cell size was decreased by 22.02–43.73% in the floral organs and by 18.54–42.94% in the berries of the POS1 -silenced mutants ( Supplementary Table 3 ). Both floral and berry cells of all 35S:POS1 transgenic Physalis plants were significantly bigger ( P ≤1.82E−25, Fig. 5c ; Supplementary Figs 13–15 ). The increase in size of these cells was 24.33–48.64% as compared with those of the WT ( Supplementary Table 3 ). However, the cell numbers were comparable in all cases ( Supplementary Fig. 16 ), suggesting that the increase in size was due to cell expansion rather than increase in the number of cells. In addition to increase in cell size, we also observed other phenotypic features such as an increase in leaf size, stem thickness and dry biomass in 35S:POS1 plants as compared with WT ( Supplementary Fig. 17 ; Supplementary Table 3 ). Thus, POS1 proteins promote cell expansion and organ size. 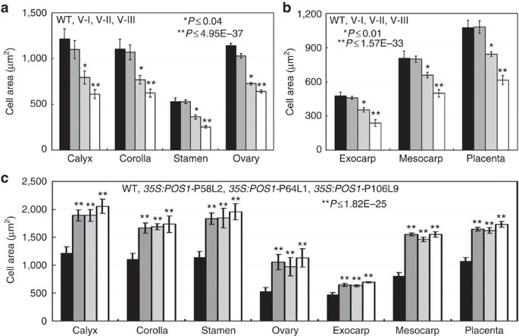Figure 5: POS1 proteins act as promoters of cell expansion. (a,b) Reduction of cell size in the VIGS-mediatedPOS1-P106-silenced mutants. (a) Cell-size variation of floral organs as indicated. (b) Cell-size variation in different areas of the median transverse section 3 days after fertilization of the berry. From left to right: WT (black column), V-I (dark-grey column), V-II (light-grey column) and V-III (empty column). (c) Cell-size variation in indicated organs of thePOS1overexpressors. Black column is for WT; grey columns are for35S:POS1-P58L2 and35S:POS1-P64L1; empty column is for35S:POS1-P106L9. Error bars are s.d. AllP-values are based on the two-tailedt-test. Compared with WT, the * indicates a significant difference (P<0.05), and the ** indicate a significant difference (P<0.01). For images, seeSupplementary Figs 12–15. Figure 5: POS1 proteins act as promoters of cell expansion. ( a , b ) Reduction of cell size in the VIGS-mediated POS1 -P106-silenced mutants. ( a ) Cell-size variation of floral organs as indicated. ( b ) Cell-size variation in different areas of the median transverse section 3 days after fertilization of the berry. From left to right: WT (black column), V-I (dark-grey column), V-II (light-grey column) and V-III (empty column). ( c ) Cell-size variation in indicated organs of the POS1 overexpressors. Black column is for WT; grey columns are for 35S:POS1 -P58L2 and 35S:POS1 -P64L1; empty column is for 35S:POS1 -P106L9. Error bars are s.d. All P -values are based on the two-tailed t -test. Compared with WT, the * indicates a significant difference ( P <0.05), and the ** indicate a significant difference ( P <0.01). For images, see Supplementary Figs 12–15 . Full size image POS1 encodes an AP2-domain protein We isolated the full-length POS1 locus of POS1 -P58, POS1 -P64, POS1 -P59 and POS1 -P106 from the three-group representatives (P58, P64 and P59) in P. philadelphica and P. floridana P106. Blast analyses suggested that the closest homologue of the POS1 gene was the SlCRF3 from tomato. Therefore, we reconstructed the neighbours of the POS1 in Physalis and SlCRF3 in tomato. The upstream gene was found to encode the putative ethylene-responsive transcription factor 1b, and the downstream gene putatively encodes the beta subunit of the pyridoxal phosphate-dependent enzyme ( Fig. 6a ). Conservation at this genomic region suggested that the local microsynteny was well maintained between Solanum and Physalis . Moreover, they were phylogenetically clustered together closely ( Supplementary Fig. 18a ); thus, these POS1 alleles are the putative orthologues of tomato SlCRF3 . They were found to encode a putative regulatory protein with double CRF (cytokinin response factor)-AP2 (APETALA2) domains ( Fig. 6a ; Supplementary Fig. 18a ). Using POS1 as a query, a comprehensive survey of the available sequence databases was conducted (Methods). Our results suggested that the POS1 -like genes were found only in Solanaceous plants, which accounts for their unique origin in the family, Solanaceae. Phylogenetic analyses revealed that POS1 proteins might have originated from a protein with one CRF-AP2 domain within Solanaceae ( Supplementary Fig. 18a ). Southern blot analysis showed that this gene is a single-copy gene that encodes POS1 having two CRF-AP2 domains in a Solanaceous genome ( Supplementary Fig. 18b,c ). The SlCRF3 expression responds to different stresses; however, its function is yet unknown [26] . The large protein family of AP2-like transcription factors is involved in multiple biological processes such as response to abiotic stresses, floral organ identity and seed size [27] . POS1 shared a similar expression pattern with the Arabidopsis AP2 (ref. 28 ), and its putative orthologues in Antirrhinum majus [29] , Zea mays [30] and Oryza sativa [31] . However, POS1 did not specify floral organ identity but controlled the floral organ size, berry size and seed size in tomatillo. The identified regulators of organ size usually exert their roles by orchestrating the two processes of cell division and cell expansion [4] , [5] , [6] . However, our work suggests that POS1 mainly promotes cell expansion. 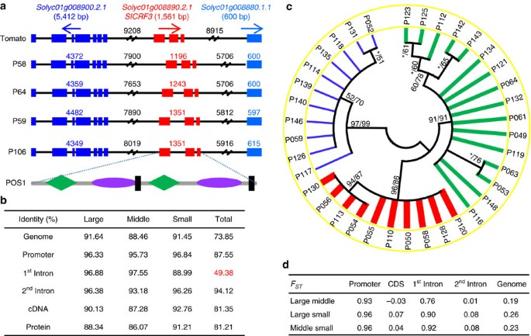Figure 6:Molecular characterizations reveal the role of thePOS1genes in tomatillo population differentiation. (a) The schematic structure of thePOS1genes. ThePOS1genes and the neighbour genes were isolated fromP. philadelphica(P58, P64 and P59) andP. floridana(P106), designated asPOS1-P58,POS1-P64,POS1-P59 andPOS1-P106, respectively. They shared the upstream gene Solyc01g008900.2.1 and the downstream gene Solyc01g008880.1.1 withSlCRF3(Solyc01g008890.2.1), thus they showed local microsynteny withSlCRF3in tomato. Introns are indicated by vertical black lines. The arrows indicate the direction of the open-reading frames indicated. The schematic diagram of POS1-like protein structure is given below. Green rhombus represents the CRF domain, and blue oval is for the AP2 domain. Black box stands for a putative MAP kinase phosphorylation site. (b) Sequence identity and variation of the tomatilloPOS1genes. The identity of the first intron is highlighted in red. (c) The sequences of thePOS1genes differentiated the collected tomatillo accessions into three groups with different berry sizes. The bootstrap value is given above each branch. The blue, green and red branches indicate the groups of the small, intermediate and large berries, respectively. (d) TheFSTvalue of different regions of thePOS1genes in tomatillo population differentiation. Figure 6: Molecular characterizations reveal the role of the POS1 genes in tomatillo population differentiation. ( a ) The schematic structure of the POS1 genes. The POS1 genes and the neighbour genes were isolated from P. philadelphica (P58, P64 and P59) and P. floridana (P106), designated as POS1 -P58, POS1- P64, POS1 -P59 and POS1 -P106, respectively. They shared the upstream gene Solyc01g008900.2.1 and the downstream gene Solyc01g008880.1.1 with SlCRF3 (Solyc01g008890.2.1), thus they showed local microsynteny with SlCRF3 in tomato. Introns are indicated by vertical black lines. The arrows indicate the direction of the open-reading frames indicated. The schematic diagram of POS1-like protein structure is given below. Green rhombus represents the CRF domain, and blue oval is for the AP2 domain. Black box stands for a putative MAP kinase phosphorylation site. ( b ) Sequence identity and variation of the tomatillo POS1 genes. The identity of the first intron is highlighted in red. ( c ) The sequences of the POS1 genes differentiated the collected tomatillo accessions into three groups with different berry sizes. The bootstrap value is given above each branch. The blue, green and red branches indicate the groups of the small, intermediate and large berries, respectively. ( d ) The F ST value of different regions of the POS1 genes in tomatillo population differentiation. Full size image Some organ-size regulators are characterized in plants [5] , [13] , [32] , [33] . However, few were proven to be involved in the natural variation of the size of certain organs. Several of the resolved loci alter the encoded protein sequence, thus, either the protein is functionally altered, or it becomes non-functional, and the resulting allelic polymorphisms can explain the origin of natural variation [34] , [35] , [36] , [37] , [38] , [39] , [40] , [41] . Nonetheless, substantial natural variation exists in gene expression within and among natural populations, and this quantitative variation is also important in the evolution of natural variation [36] , [42] . We comprehensively evaluated the role of the POS1 sequence variation in the observed variations of reproductive organ size. Regulatory variation at POS1 correlates to organ sizes Variation in the coding region of a gene is often associated with functional divergence. To evaluate this, we sequenced the POS1 cDNA from tomatillos, and found that the 37 sequences obtained shared 81.4% identity with nucleotides and 81.2% identity with their encoded proteins. Multiple protein alignments revealed 244 polymorphisms ( Supplementary Fig. 19 ). Among these sites, 14 were detected to correlate to size variation in one or two traits of flower size, fruit weight and 100-seed weight; however, only one site (position 401) was significantly associated with the size co-variation of the three quantitative traits ( P ≤0.04, Supplementary Table 4 ). The evolutionary role of the protein sequence divergence needs further investigation. However, similar observations of organ-size variation in our transgenic Physalis (P106) analyses with different POS1 alleles suggested that POS1 proteins might have maintained a similar function during evolution. Therefore, altering POS1 expression might be key to the evolution of diversities in reproductive organ size in tomatillos. Recruitment of a POS1 function for reproductive organ size in tomatillos might have occurred in response to mutations in a trans -acting regulator or to changes in the cis -regulatory elements of the POS1 gene itself. Association analyses in the F 2 population suggested that a local cis -regulatory element might control POS1 expression. Therefore, we sequenced the POS1 genes from all tomatillo accessions. Gene structure of intron–exon arrangement was found to be quite conserved as shown for POS1 -P58, POS1 -P64 and POS1 -P59 ( Fig. 6a ); however, the POS1 sequences of tomatillos could be divided into three subgroups, corresponding exactly to the three groups defined for different reproductive organ sizes ( Fig. 6b,c ). Like cDNA (exons), the promoters and the second introns among these accessions shared a relatively high identity while the first intron from different accessions had a 49.38% identity in sequences ( Fig. 6b ). The exons and the second intron sequences could not differentiate the population ( Supplementary Fig. 20a,c ); however, both promoters and the first introns could do so as could the whole-gene sequences ( Fig. 6c ; Supplementary Fig. 20b,d ). Furthermore, F ST values of both promoter and the first intron instead of the exons and the second intron suggests a complete differentiation of the tomatillo population structure ( Fig. 6d ) that precisely corresponds to the three different size groups ( Fig. 1 ; Supplementary Table 1 ). Regulatory alterations in a pre-existing gene play an important role in the evolution of phenotypic variations. Thus, the regulatory variations in the POS1 alleles leading to different expression levels affect the natural variations in the size of reproductive organs. Sequence analysis of the promoters and introns of POS1 showed that the variation in the promoter sequences determined the populations, which could be differentiated into three groups on the basis of berry size having small, intermediate and large berries ( Supplementary Fig. 20d ), but no notable difference accounting for the differential POS1 expressions was found in the polymorphic promoters. The second introns were relatively conserved in sequence and length ( Supplementary Fig. 21a ) while significant differences in sequence and length of the first introns were observed in POS1 of P. philadelphica ( Fig. 7a ; Supplementary Fig. 21b ). Further studies revealed that the first intron consisted of a variable region and a conserved region (113–122 bp; Supplementary Fig. 21b ). The variable regions of 34, 91 and 341 bp in large, immediate and small berry groups, respectively, were composed of one, two and three copies of a 37-bp repeat with a consensus as 5′-GTaCTGaaaCTtTCTTAGAGTCAGCAgTTCCGTCTtt-3′ ( Fig. 7b ). Blast analysis did not reveal any putative conserved regulatory motifs. The first intron length was mainly determined by the copy number of the 37-bp repeat. The alleles from the large berry group with a high POS1 expression maintained one repeat, the alleles from the immediate berry group with a moderate POS1 expression kept two repeats and the alleles from the small berry group with a low POS1 expression harboured three repeats ( Fig. 7a ; Supplementary Figs 1 and 21b ). Obviously, the first intron length and its copy number of the 37-bp repeat were negatively correlated with POS1 expression from three organ-size groups in tomatillos ( Supplementary Table 2 ). As the first introns became shorter due to a decrease in copy number of the 37-bp repeats, a higher gene expression resulted in a simultaneous increase in berry size, seed size and flower size in tomatillos. Therefore, the first intron of the gene itself is likely the local cis -element controlling the POS1 expression levels. 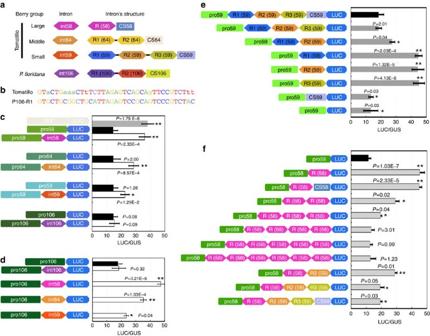Figure 7:The first introns and 37-bp repeats of the tomatilloPOS1alleles determine the gene expression levels. (a) Berry-size groups correspond to different introns in tomatillos. The intron (int) structure was shown fromPOS1-P58 (int58, large berry),POS1-P64 (int64, intermediate berry) andPOS1-P59 (int59, small berry). An intron indicated by different colours and ending with the accession number includes the 37-repeats (Rs) and the conserved sequences (CS). The intron structure ofP. floridana(POS1-P106) was also given. (b) The composition of the 37-bp repeats. Tomatillo-type repeat consensus was summarized from the 75 repeats of 37 accessions. The divergent nucleotide is given in small and the consensus in capital. The first 37-repeat inPOS1-P106 (P106-R1) that shared the highest identity with the tomatillo-type was aligned with the tomatillo-type consensus. (c–f) Transient activation assays of the luciferase (LUC) reporter gene driven by differentPOS1regulatory regions. (c) Relative LUC activity driven by differentPOS1promoters and their fusions with the first intron of their own as indicated.35S:LUCwas used as a control and its LUC activity is indicated by a grey column. (d) Relative LUC activity driven by thePOS1-P106 promoter fusing to the first intron of thePOS1alleles as indicated. (e) Regulatory role of the 37-bp repeats from thePOS1-P59. (f) Copy-number variation of the tomatillo-type 37-bp repeats regulates gene expression. Three independent experiments were performed in each case. Mean expression is presented. The error bars represent the s.d. TheP-values of the two-tailedt-test compared with each control (black column) indicated are given. The * indicates a significant difference (P<0.05), and the ** indicate a significant difference (P<0.01). Figure 7: The first introns and 37-bp repeats of the tomatillo POS1 alleles determine the gene expression levels. ( a ) Berry-size groups correspond to different introns in tomatillos. The intron (int) structure was shown from POS1 -P58 (int58, large berry), POS1 -P64 (int64, intermediate berry) and POS1 -P59 (int59, small berry). An intron indicated by different colours and ending with the accession number includes the 37-repeats (Rs) and the conserved sequences (CS). The intron structure of P. floridana ( POS1 -P106) was also given. ( b ) The composition of the 37-bp repeats. Tomatillo-type repeat consensus was summarized from the 75 repeats of 37 accessions. The divergent nucleotide is given in small and the consensus in capital. The first 37-repeat in POS1 -P106 (P106-R1) that shared the highest identity with the tomatillo-type was aligned with the tomatillo-type consensus. ( c – f ) Transient activation assays of the luciferase (LUC) reporter gene driven by different POS1 regulatory regions. ( c ) Relative LUC activity driven by different POS1 promoters and their fusions with the first intron of their own as indicated. 35S:LUC was used as a control and its LUC activity is indicated by a grey column. ( d ) Relative LUC activity driven by the POS1 -P106 promoter fusing to the first intron of the POS1 alleles as indicated. ( e ) Regulatory role of the 37-bp repeats from the POS1 -P59. ( f ) Copy-number variation of the tomatillo-type 37-bp repeats regulates gene expression. Three independent experiments were performed in each case. Mean expression is presented. The error bars represent the s.d. The P -values of the two-tailed t -test compared with each control (black column) indicated are given. The * indicates a significant difference ( P <0.05), and the ** indicate a significant difference ( P <0.01). Full size image The first intron of POS1 regulates gene expression We next evaluated the regulatory role of the first intron in gene expression using the reporter gene, luciferase (LUC), introduced in Physalis protoplasts. A 35S:GUS construct was co-transformed as a reference in the well-established methodology [43] , [44] , and the measurement of LUC/GUS was presented as the gene expression level of the corresponding regulatory sequences. The results indicated that the POS1 promoters from both tomatillos and P106 drove similar expression levels ( Fig. 7b ). However, unlike the first intron from POS1 -P106, the tomatillo-type first introns significantly enhanced gene expression once they fused with any POS1 promoters tested ( P ≤1.29E−2; Fig. 7c,d ). Moreover, short first introns, such as POS1 -P58, could activate the strongest gene expression, while long first introns, such as POS1 -P59, activated the lowest gene expression. Length determination of the first introns by the occurrence of the 37-bp repeats ( Fig. 7a ) suggests that the 37-bp repeats may have an important role in the regulation of gene expression. We manipulated the 37-bp repeats (see Methods, Fig. 7e,f ), that decreased the copy number from three to one. The single tomatillo-type 37-bp repeat could enhance gene expression significantly ( P ≤0.03) while increasing the copy number of the repeats to two and three significantly attenuated the gene expression ( Fig. 7e,f ). However, this attenuated gene expression was higher than that of the promoter itself ( P ≤0.04). Moreover, when the copy number was beyond 3, the enhancing effects on gene expression were completely abolished ( Fig. 7f ). Thus, the regulatory role of tomatillo-type 37-bp repeats in gene expression in protoplasts mimicked the naturally evolved functioning patterns of the POS1 expression observed in tomatillos. The first intron and the 37-bp repeat variants of POS1 -P106 had lost the ability to enhance gene expression ( Supplementary Fig. 22 ), and they were apparently diverged in sequences from the tomatillo-type repeats that were highly conserved ( Fig. 7b ; Supplementary Fig. 23a,b ). These results suggest that the enhancing effect requires sequence specificity. Thus, the evolution of such a conserved 37-bp repeat and its copy-number variation in the first intron of the POS1 genes is largely responsible for dosage expressions of this gene in tomatillos. POS1 function in organ size is specific to Physalis species Variations in organ size are common among natural populations, and they can affect crop yield. Fruit (grain) size is a prime breeding target of crop breeders. Grain size-regulating genes (GS), such as GS3 and GS5 that cause a large difference in grain size were characterized in rice [36] , [45] , [46] , [47] . GS3 and GS5 are strongly associated with natural variation of grain size [36] , [45] . In Solanum , FW2.2 , FAS and LC , as negative regulators, account for >80% of the berry size difference between WT tomato and its cultivated relatives [13] , [17] , [18] . A few characterized regulators could explain an exaggerated difference in the floral organ size [48] , [49] , [50] . However, molecular genetic mechanism of co-variation of floral organs and post-floral organs (fruits and seeds) is not well studied in plants. The regulatory role is achieved through altering the cis -regulatory elements in the first intron of POS1 alleles and may form the basis of the genetic architecture underlying this co-variation of reproductive organs. Introns can regulate gene expression in plants [17] , [51] , [52] , [53] and animals [54] , [55] . Therefore, copy-number variation in the 37-bp repeat in the ‘first intron of the POS1 genes’ probably affected the size variation in the reproductive organs of P. philadelphica ( Supplementary Table 2 ). Thus, the altered gene expression mechanism can be associated with co-variation of reproductive organ size in plants. Further investigation in the interspecies of the non-tomatillo Physalis species revealed a weak correlation between the intron length, and expression of the POS1 alleles, and floral organ size. However, the copies of the 37-bp composition had no correlation with gene expression and berry size ( Supplementary Tables 5 and 6 ). Unlike the tomatillo-type repeats, they shared a 97.8% identity in sequences with a low nucleotide diversity ( π =0.026). The non-tomatillo 37-bp repeats shared a low identity ( ca . 70%) with a high nucleotide diversity ( π =0.386) ( Supplementary Fig. 23 ). Moreover, the POS1 sequences did not give a clear phylogenetic relationship among Physalis species ( Supplementary Fig. 24 ). Furthermore, the SlCRF3 genes, which are the putative orthologues of the POS1 genes, featured nearly identical gene sequences between S. lycopersicum and S. pimpinellifolium , and their expression was not similarly regulated as those in Physalis ( Supplementary Fig. 25 ). Therefore, the POS1-like function controlling the reproductive organ size might be specific to Physalis species, such as tomatillos. Different tomatillo cultivars produce berries of various sizes; however, both the wild and small tomatillos were harvested by the farmers for the market [23] . Although size may not have been a preferred trait initially, it might be an important agronomic trait to meet the growing demand of tomatillos for their medicinal and culinary uses. Our study shows that the genetic variation in the polymorphic POS1 alleles controls the natural variation in berry size ( Supplementary Figs 19 and 21 ); thus, this knowledge can be utilized in the domestication of tomatillos based on their size. In summary, our results show that POS1 mainly acts as a promoter of cell expansion. Changes in the first intron of the POS1 genes are recruited to co-regulate the size of flowers, berries and seeds in tomatillos. Our work shows that the evolution of size variation in organs can be attributed to rare genetic variations in the intron, further highlighting the importance of variations in transcript abundance in domestication and evolution of species. Further studies can investigate the impact of these regulatory changes on the overall yield and the effect of enhanced cell size (due to POS1) on organ size in tomatillo. Plant materials P. floridana [19] , S. lycopersicum and S. pimpinellifolium were obtained from the Seed Bank of the Max Planck Institute for Plant Breeding Research (MPIZSB). Information of other Physalis resources is available in Supplementary Tables 1 and 5 . These plants were grown in 2009, 2010 and 2012 at the Institute of Botany, Chinese Academy of Sciences (IBCAS, Beijing, China). The seedlings were cultivated in a greenhouse under long-day conditions (temperature 25–28 °C, illumination 16 h) until flowering. For a better fruiting rate, they were moved to the experimental fields during the summer. The roots, stems, leaves, mature flowers and developing berries of these species or transgenic plants involved (as indicated in each experiment) were harvested, immediately frozen in liquid nitrogen and stored at −80 °C. Three independent biological samples were collected, and total RNA was isolated using the TRIzol Reagent (Invitrogen). The genomic DNA from leaves was extracted using the Plant Genomic DNA Extraction Kit (GenStar Biosolutions). Visualization of chromosome number and POS1 copy number Root-tip samples from 1-week-old seedlings of tomatillos were collected to count the chromosome number. Samples were fixed in Carnoy’s fixative (ethanol:glacial acetic acid 3:1) at room temperature for at least 4 h before storing at –20 °C. Chromosome spreads were then stained with 4′,6-diamidino-2-phenylindole and the slides were examined under a fluorescence microscope (Axioskop40 with HBO100, Zeiss). The chromosomes of 15 cells were counted, and the mean and s.d. were calculated. Southern blotting analyses were performed to evaluate the copy number of POS1 gene in Physalis . Genomic DNAs (10 μg) of P106, P58, P64 and P59 were digested using BamH I, Hind III, EcoR I and EcoR V (TaKaRa, Dalian, China) as indicated. DNA gel blots were conducted by capillary transfer with 20 × saline-sodium citrate on a positively charged nylon membrane (GE Healthcare, Uppsala, Sweden). Thereafter, the 480-bp POS1 cDNA fragments were randomly labelled with digoxigenin (DIG)-dUTP and hybridization was performed using the DIG high prime DNA labeling and detection starter kit II, version 13 (Roche, Mannheim, Germany). The DIG-labelled probe was detected by chemiluminescence and then the membrane was exposed to an X-ray film. Gene isolation and sequencing analyses 5′- and 3′-rapid amplification of cDNA ends (RACE, Roche) were performed based on the Pp30 fragment obtained previously [20] . PfCRF7 and PfCRF8 in P. floridana , which shared the most similarity with Pp30 (or POS1 ), were isolated based on their putative orthologues of SlCRF7 and SlCRF8 in Solanum . PCR products were purified using the High Pure PCR Product Purification Kit (Roche). The fragments were cloned into the pGEM-T easy Vector (Promega) and transformed into competent Escherichia coli DH5α cells (Tiangen) by electroporation. Plasmid DNA was extracted using the AxyPrep Plasmid Miniprep Kit (Axygen). Sequencing was commercially done by BGI (Beijing Genomics Institute). The cDNA and genomic DNA sequences were obtained using RT–PCR or genomic PCR, respectively. Primers used for sequence isolation of the POS1 genes are available in Supplementary Table 7 . The similarity among these sequences was analysed using the software DNAMAN. Identification of the POS1 homologous genes To identify homologues, POS1 full-length sequences were used as a query to search in a wide variety of available genome sequencing data in NCBI ( http://blast.ncbi.nlm.nih.gov/Blast.cgi ), Phytozome ( http://www.phytozome.net/search.php ) and Sol Genomics Network ( http://solgenomics.net/tools/blast/index.pl ) including 28 vertebrates, 16 invertebrates, 19 protozoa, 118 plants and 17 fungi, all together 198 species. The consensus sequences of CRF and APETALA2 (AP2) domains were used to do BLAST searches separately in these databases. Proteins identified by BLAST search algorithms were considered as potential homologues when amino-acid identity was above 40% over the stretch of full-length sequences. The Pfam ( http://pfam.janelia.org/ ) and SMART ( http://smart.embl-heidelberg.de/ ) databases were employed to detect conserved domains with POS1-like protein candidates. Sequence logos were generated using the WebLogo software ( http://weblogo.berkeley.edu/logo.cgi ) [56] . Phylogeny of the POS1-like proteins Multiple sequence alignments were performed by the Clustal X (v1.81) [57] . The sequences were adjusted manually using BioEdit (v7.0.5) where necessary so as to optimize the alignment [58] . The maximum likelihood phylogenetic tree of the POS1 closely related proteins was constructed using PhyML (v3.0) under the LG amino-acid substitution model, with 100 replicates of bootstrap analysis, estimated gamma distribution parameter and optimized starting BIONJ tree [59] , [60] . The sequence information for the POS1-like phylogenetic tree is available in Supplementary Table 8 . The obtained phylogenetic trees were visualized by TreeView1.6.6 tool with a 50% threshold of branch value [61] . Phylogenetic analyses of Physalis species On the basis of the POS1 cDNA and gene sequences (the first intron, the second intron and promoter) that were isolated in the present work, the phylogenetic trees of the collected Physalis were constructed using the neighbour-joining distance method and the maximum parsimony method with 1,000 replicates of bootstrap analysis by the MEGA version 5.0 (ref. 62) [62] . The obtained phylogenetic trees were visualized by TreeView1.6.6 tool with a 50% threshold of branch value [61] . qRT–PCR analyses About 2.0 μg total RNA was used for cDNA synthesis with the SuperScript II Reverse Transcriptase (Invitrogen). Assays were performed with 1.0 μl cDNA, diluted two folds, using the SYBR Premix Ex Taq (TaKaRa). The quantification method (Delta-Delta CT) was used to evaluate variation between replicates [63] . The PFACTIN gene was used as an internal control to normalize the data. PCR conditions consisted of an initial denaturation step at 95 °C for 3 min, followed by 40 cycles at 95 °C for 30 s, 60 °C for 1 min and 72 °C for 30 s and a final extension at 72 °C for 5 min. Primers used for qRT–PCR are listed in Supplementary Table 7 . Amplification efficiencies of the gene-specific primers were between 95 and 105%. POS1 mRNA in situ hybridization A 284-bp POS1 -P106-specific fragment was cloned into the pGEM-T easy Vector System (Promega) to synthesize the sense and antisense probes with a linear plasmid according to the Digoxigenin (DIG) RNA labeling kit manual (Roche). Primers used for PCR and probe synthesis are listed in Supplementary Table 7 . Tissues were fixed overnight (12 h) in RNase-free formalin–glacial acetic acid–alcohol. Samples were dehydrated in a graded ethanol series and embedded in Paraplast Plus (Sigma). Hybridization procedures were described previously [64] . Briefly, the tissue sections were pretreated including the deparaffinized and rehydrated processes. Hybridizations were performed at 45 °C overnight. Hybridization signal was detected by chemiluminescence with NBT/BCIP stock solution (Roche). Images were examined under a fluorescence microscope (Axioskop40 with HBO100, Zeiss). Transient LUC activity assays To produce the LUC (luciferase) reporter gene constructs driven by the POS1 promoter ( POS1 -P58, POS1 -P64, POS1 -P59 and POS1 -P106), 1.8-kb fragments upstream of the translational start site were amplified from each genome. Hind III- and BamH I-cutting sites were in-frame introduced to the 5′- and 3′-ends, respectively. The expected DNA fragments were cut with Hind III and BamH I and ligated into the YY96 vector [65] . To make promoter-intron chimeric constructs, the promoter (using the allele-specific forward and reverse primers in which the Hind III- and Nde I Sac I-cutting sites were introduced, respectively) and the first intron (using the allele-specific primers in which the Nde I- and BamH I Sac I-cutting sites were introduced in the forward and reverse primers, respectively) were amplified and inserted into the pGEM-T Easy (Promega), respectively. Both sequenced constructs were cut with Nde I and Sac I, and then the first intron was precisely ligated with the promoter. The chimerical promoter-intron fragments were obtained via cutting with Hind III and BamH I and were ligated into the YY96 vector. To produce the LUC reporter gene driven by the POS1 promoter with different copy number of the 37-bp repeat, the promoter (using allele-specific primers that harbour the Hind III-cutting site in the forward primers and Nde I- and Sac I-cutting sites in the reverse primers) and the 37-bp repeat were amplified (using the primers of R-F1with the Nde I-cutting site and R-R1 with BamH I Sac I-cutting sites), respectively, and were inserted into the pGEM-T Easy (Promega). The two products were cut with Nde I and Sac I, and then the repeats were ligated with the promoter in the pGEM-T Easy. The POS1 promoter—the repeat was cut with Hind III and BamH I and ligated into the YY96 vector. The multiple repeats were introduced with the primer combination of R-F2 and R-R2 (or R1-R1) with similar restriction endonuclease-cutting sites in the R-F1 and R-R1, respectively. Primers used for reporter gene constructs are shown in Supplementary Table 7 . Protoplast preparation of P. floridana (P106) and transient expression assays were performed as described previously [43] , [44] . Briefly, each obtained reporter plasmid and 35S:GUS internal control were co-transformed into protoplasts. For LUC assays, plastid combinations of various N- and C-terminal LUC fusions were co-transformed with the 35S:GUS internal control. The protoplasts were pelleted and resuspended in 1 × cell culture lysis reagent (Promega). The GUS fluorescence was measured using a Modulus luminometer/fluorometer with a UV fluorescence optical kit (Promega). The LUC activity was detected with a luminescence kit using LUC assay substrate (Promega). The relative reporter gene expression levels were expressed as the LUC/GUS ratios. Construction of a F 2 -segregating population The tomatillo accessions P58 and P64 that show marked polymorphisms in reproductive organ sizes were crossed for a F 2 population consisting of 242 progeny. To evaluate the population, total DNA from P58, P64, F 1 hybrid and F 2 progeny were subjected to PCR. Two polymorphic DNA markers were developed based on MPF2 [19] and POS1 ( Pp30 ) [20] . Primers used for molecular segregation and linkage analyses are listed in Supplementary Table 7 . Polymorphisms of the PCR products were visualized on 1.2% agarose gels. Genotype of each individual at MPF2 or POS1 locus was recorded as homozygous P58 type or P64 type, and heterozygous P58-P64 type. Physalis transgenic analyses The open-reading frame of POS1 -P106, POS1 -P58 and POS1 -P64 was inserted into the plant binary vector pBAR for making the overexpression construct. P. floridana P106 was used for transformation as described previously [19] . Briefly, cotyledons were used as explants, and Agrobacterium tumefaciens strain LBA4404 was used for transformation. T 1 transgenic plants were selected in half-strength MS (Murashige and Skoog) medium containing phosphinothricin (5.0 mg l −1 ) and 5.0 mg l −1 Claforan (Sigma-Aldrich). These transgenic P106 plants were grown in a greenhouse under long-day conditions and characterized by BAR (phosphinothricin- N acetyl transferase) gene genomic PCR, POS1 by RT–PCR and phenotypic analyses. T 2 plants derived from the positive T 1 plants were screened on MS medium containing phosphinothricin. The survivors were transplanted in nutrient soil mixed vermiculite (volume=3:1) in a growth chamber under long-day conditions (temperature 22–25 °C, illumination 16 h) for further phenotypic analyses and genotyping RT–PCRs. The WT plants that were germinated on MS medium were transplanted and used as controls. During cultivation, half-strength MS solution without sucrose was irrigated in the pots. Primers used for making constructs and genotyping of transgenic plants are listed in Supplementary Table 7 . VIGS analysis 480-bp of the 3′-end of the POS1 -P106 cDNA was introduced into the TRV-mediated VIGS vectors as a previous description [66] . Briefly, the TRV-mediated VIGS vectors were infiltrated into 2-week-old Physalis seedlings. Primers used for VIGS constructs are listed in Supplementary Table 7 . The PfPDS -VIGS and PfP12 -VIGS plants were included as controls. VIGS analyses were performed in P. floridana (P106). The cultivation conditions were same as those used for other transgenic plants. Analysis of morphological traits The size of the mature flower was represented by the length between the receptacle and the tip of mature flowers. The final size of calyx, corolla and stamen was measured by the length between the receptacle and the tip of sepal, petal or stamen when the flower was fully open. Ovary size was defined by the distance from the receptacle to the place that the stigma was located in the mature flowers. Fresh mature berry size was defined either by the weight or volume. Berry volume was determined by immersing a berry into a measuring cup containing water; the elevation of the water volume was recorded as the berry volume. Seed number per mature berry was counted, and 100-seed weight was balanced. For each plant/accession, the size of 15–60 mature flowers and 10–100 mature berries was quantified. Three-month-old plants were dried at 65 °C for dry biomass measurement. The floral images were taken using a microscope equipped with a Nikon camera. Leaf size and stem section area were measured using AxioVision Release 4.7.2. Scanning electron microscopy Flowers and fruits were immediately fixed in formaldehyde acetic acid solution (3.7% formaldehyde, 50% ethanol and 5% acetic acid) for 24 h and then dehydrated in a graded ethanol series. The dehydrated materials were critical-point dried in liquid CO 2 and mounted on metallic stubs. The mounted materials were shadowed with gold and then applied to the scanning electron microscope (Hitachi S-800). Histological analysis For paraffin sectioning, the berries (about 3 days after fertilization) and stems from 1-week-old seedlings were fixed overnight at 4 °C in FAA solution (formalin: glacial acetic acid: alcohol, 90: 5: 5, v/v/v); these were dehydrated in a graded ethanol series, and then embedded in paraffin wax (Sigma). Tissue sections were cut with a microtome, and stained with safranin-fast green [67] , which dyed the lignified secondary cell walls of the vessels and the endodermal cells red, and the living cells green. The slides were examined and photographed under the microscope (Axioskop40 with HBO100, Zeiss). The cell number of the median transverse section of berries was counted, and the cell area was measured using AxioVision Release 4.7.2. The mean cell number and cell size were estimated as previously described [13] , [14] . Briefly, cell number was calculated from the cell size counted per unit area (1 mm 2 ) measurements (excluding developing seeds). The mean stem cell size measurement excluded vascular bundles. Statistical analyses Distribution of flower size, berry size (weight and volume), seed weight and gene expression in the F 2 -segregating population was evaluated using the SPSS 15.0. Statistical analysis of the mean value, correlation coefficient ( R ), χ 2 -test, variance and normal distribution were tested using SPSS 15.0. Genetic contribution was evaluated using the MapQTL 5.0 program. PVE (phenotypic variation explained %)= V g/ V p × 100%. V g means genetic variance and V p means phenotypic variance. Multiple-QTL model was tested for linkage analyses. LOD (likelihood of odd)=3.0. Significance evaluation ( P -values) was evaluated using the two-tailed Student’s t -test. Association between the variation in amino-acid sites and quantitative traits (fruit weight, 100-seed weight and flower size) was analysed using one-way analysis of variance of SPSS 15.0. Population differentiation was estimated using Wright’s F ST statistics, and nucleotide diversity ( π ) of the 37-bp repeats was calculated using DnaSP version 5. Accession codes: Isolated sequences annotated using the BLAST program have been deposited in GenBank/EMBL/DDBJ nucleotide core database under the accession codes KJ754713 to KJ754816 . How to cite this article: Wang, L. et al. Regulatory change at Physalis Organ Size 1 correlates to natural variation in tomatillo reproductive organ size. Nat. Commun. 5:4271 doi: 10.1038/ncomms5271 (2014).